Potential climate engineering effectiveness and side effects during a high carbon dioxide-emission scenario The realization that mitigation efforts to reduce carbon dioxide emissions have, until now, been relatively ineffective has led to an increasing interest in climate engineering as a possible means of preventing the potentially catastrophic consequences of climate change. While many studies have addressed the potential effectiveness of individual methods there have been few attempts to compare them. Here we use an Earth system model to compare the effectiveness and side effects of afforestation, artificial ocean upwelling, ocean iron fertilization, ocean alkalinization and solar radiation management during a high carbon dioxide-emission scenario. We find that even when applied continuously and at scales as large as currently deemed possible, all methods are, individually, either relatively ineffective with limited (<8%) warming reductions, or they have potentially severe side effects and cannot be stopped without causing rapid climate change. Our simulations suggest that the potential for these types of climate engineering to make up for failed mitigation may be very limited. The realization that despite all mitigation efforts to reduce CO 2 emissions atmospheric CO 2 concentrations are still rapidly increasing and closely follow the IPCC’s high emission scenario [1] has led to an increasing interest in climate engineering as a potential means of preventing the potentially unacceptable consequences of global warming [2] , [3] . Evaluating the potential effectiveness and risks of different climate engineering methods prior to any large-scale field experiments is an important first step in informing scientists and society if, and how, further research or physical experimentation should be done [4] . Besides providing information regarding potential opportunities and risks, theoretical research has also proven to be a useful way to learn about the climate system. While there is a growing body of literature on individual methods, comparisons among different studies are difficult to make when the studies have been conducted with different models and climate change scenarios [3] . A previous comparison of the radiative forcing potential of different climate engineering methods [5] addressed the question of how efficient the methods are at preventing global warming. However, the analytical methodology that was used did not allow for the quantification of side effects and the possible feedbacks in the climate system that may cause a method to be more or less effective than predicted. Earth system models can be used to better evaluate the effectiveness, side effects and climate feedbacks of different climate engineering methods in a comprehensive way, but have not yet been used to compare different climate engineering methods. 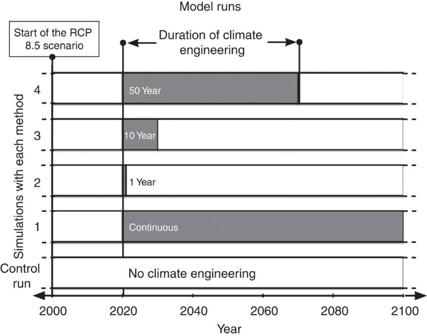Figure 1: Experimental design. The simulations performed for each climate engineering method. The control run is also depicted. The objective of this paper is to compare and assess the potential effectiveness, in terms of intended climate remediation, as well as the unintended physical and biogeochemical side effects of several climate engineering methods ( Table 1 ) during transient Earth system simulations with a high CO 2 emissions representative concentration pathway (RCP 8.5) scenario [6] ( Fig. 1 ). We employ the University of Victoria Earth system model (UVic) [7] , [8] , a model of intermediate complexity (EMIC), and investigate various climate engineering methods of different character in terms of deployment medium, spatial and temporal scales, as well as ethical, legal and cultural aspects. These methods are large-scale afforestation (AF), ocean iron fertilization (OIF), artificial ocean upwelling (OU), ocean alkalinization (OA) and solar radiation management (SRM). For simplicity, our approach for many of the methods is idealized to simulate the effects that deploying a method would have, without introducing unnecessary complexity (see Methods). Moreover, we also evaluate the methods in a manner that essentially investigates near-maximum potential effects (that is, large to global-scale deployments with an intensity as large as currently deemed feasible—see Methods). The economic, legal, political and technological feasibility of the methods are not considered here, nor are ethical aspects. Instead we focus solely on the potential atmospheric CO 2 reductions, climate impacts and the physical and biogeochemical side effects of each method. We find that even when applied continuously at scales as large as currently deemed possible, all methods are, individually, either relatively ineffective with limited warming reductions, or they have potentially severe side effects and cannot be stopped without causing rapid climate change. Our simulations suggest that the potential for these types of climate engineering to make up for failed mitigation may be very limited. Table 1 Climate engineering methods evaluated. Full size table Figure 1: Experimental design. The simulations performed for each climate engineering method. The control run is also depicted. Full size image Model trends during the RCP 8.5 climate change scenario The UVic model has recently been evaluated in several model intercomparison exercises [9] , [10] , [11] and generally has a similar response to CO 2 emission forcing as other models. Here we will briefly mention how the results of our RCP 8.5 scenario control run ( Supplementary Figs 1–3 ) compared with other models. We will also point out the trends that differ from other models since these (possible) biases need to be taken into consideration when evaluating the model’s response to climate engineering. For surface air temperature the model simulates a global mean warming of 3.1 °C by the year 2100 relative to a 1986–2005 reference period (see also Fig. 2c for warming relative to the pre-industrial period), which is within the ranges of an EMIC intercomparison (1.6–4.1 °C) [10] and the CMIP5 models (2.5–5.0 °C) [12] . Atlantic meridional overturning circulation decreases by 38% in our simulation, which is near the mean (40%) and within the range (36–44%) of 26 other models (mostly CMIP5 models) [11] . For ocean biogeochemistry a CMIP5 model intercomparison study has not yet been published so instead we have made comparisons to the Community Earth System Model (CESM1 (BGC)) RCP 8.5 scenario results [13] . By the year 2100 export production has decreased by 11% in our simulation and 13% in the CESM1 simulation. Net primary production decreases by 5.8% in our simulation and 5.7% in the CESM1 simulation. Mean ocean oxygen decreases by 7 μM in our simulation (see also Fig. 2g for the global total change in oxygen) and 10 μM in the CESM1 simulation. However, for the volume of the oxygen minimum zones (OMZ), our results are in contrast to CESM1, since our simulation shows a decrease in the size of the OMZs ( Supplementary Fig. 4 ) and theirs show an increase of 24%. Since most Earth system models have problems simulating oxygen distributions and the volume of OMZs it is difficult to determine which trend is correct [13] , [14] , [15] , although observations suggest that OMZs have been expanding in recent decades [16] . Evaluating terrestrial carbon uptake or loss is difficult since there are large differences (that is, uncertainty) in total carbon uptake between the CMIP5 models (ranging from −0.97 to 2.27 Pg C y −1 during 2006–2100), with some models predicting that the terrestrial biosphere will become a net source of carbon and other predicting that it will become a larger sink [17] . 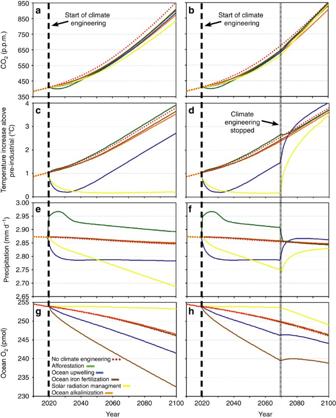Figure 2: Comparison of climate engineering method effects on key global properties. Simulated changes in globally averaged annual atmospheric CO2and surface air temperature (relative to a pre-industrial temperature of 13.05 °C) and the total amount of annual global precipitation and ocean oxygen for model runs where climate engineering was continuously deployed (a,c,eandg) and runs where it was discontinued after 50 years (b,d,fandh). The control run, with no climate engineering, is also shown. In our simulation the terrestrial biosphere becomes a larger sink with a terrestrial carbon pool in the year 2100 ( Table 2 ) that is 15 Pg C larger than the highest value reported for the CMIP5 models [17] . For soil moisture our model indicates that globally soil moisture will decrease in June, July and August and increase in December, January and February (DJF). The first result is largely consistent with CMIP5 model results [18] . However, the majority of CMIP5 models indicate that while a large proportion of the globe will have higher soil moisture in DJF an even larger proportion will have drier conditions [18] , which is inconsistent with our results. For precipitation our model does not show a global increase of 1–3% K −1 as warming occurs, which is inconsistent with most models [19] , [20] , [21] . Instead global precipitation in the model decreases by 0.3% K −1 (see also Fig. 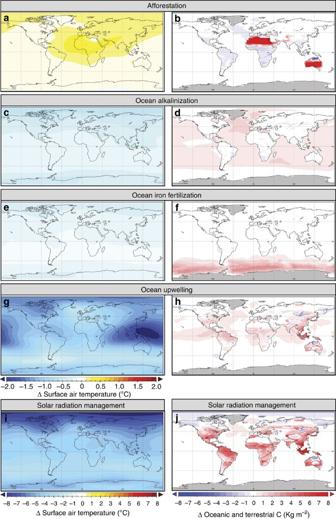Figure 3: Climate engineering method effects on temperature and carbon storage. The simulated year 2100 mean annual differences between the climate engineering runs and the control run (climate engineering run minus the control run) for surface air temperature (a,c,e,gandi) and terrestrial and oceanic carbon inventories (b,d,f,handj). Note the difference in the surface air temperature scale for solar radiation management. 2e and Table 3 for mean annual changes). This inconsistency occurs despite an increase in atmospheric water vapour of 7.4% K −1 , which is consistent with other models, observations, and in line with the Clausius–Claperyron equation [19] , [20] , [21] . The decrease in global precipitation is entirely due to a decrease in terrestrial precipitation of 3.41% K −1 since precipitation and evaporation over the ocean increase by ~1.26% K −1 , which is in good agreement with other models ( Supplementary Fig. 5 ). The decrease in terrestrial precipitation is related to the simulated sensitivity of evapotranspiration to increasing CO 2 (that is, the physiological response of plant stomata to CO 2 fertilization and its effect on water vapour loss), which results in a reduction in terrestrial evaporation of 8% K −1 . While this strong decrease in evapotranspiration is inconsistent with the general trend of other models (despite significant differences and uncertainty among them [22] ), recent research [23] has suggested that existing theory and the 13 most commonly used terrestrial biosphere models underestimate forest water-use efficiency when CO 2 increases. Figure 2: Comparison of climate engineering method effects on key global properties. Simulated changes in globally averaged annual atmospheric CO 2 and surface air temperature (relative to a pre-industrial temperature of 13.05 °C) and the total amount of annual global precipitation and ocean oxygen for model runs where climate engineering was continuously deployed ( a , c , e and g ) and runs where it was discontinued after 50 years ( b , d , f and h ). The control run, with no climate engineering, is also shown. Full size image Table 2 Climate engineering induced changes in global temperature and carbon inventories. Full size table Table 3 Climate engineering induced changes in key Earth system properties. Full size table Climate engineering method effects on temperature and CO 2 When climate engineering is deployed continuously from the year 2020 onward, atmospheric CO 2 is reduced in all of the simulations ( Fig. 2a , Table 2 ). However, these reductions are small compared with expected business-as-usual anthropogenic emissions, and atmospheric CO 2 continues to increase rapidly and still reaches more than twice the current level by the end of the century in all simulations. Those methods that have been proposed to reduce atmospheric CO 2 as a means of preventing warming, that is, carbon dioxide reduction (CDR) methods ( Table 1 ), are thus, as expected from other studies [3] , [5] , [24] , [25] , [26] , [27] , unable to prevent a 2.7–3.9 °C mean temperature increase (temperature increases by 3.8 °C with no climate engineering) in our model simulations under the RCP 8.5 emission scenario by the year 2100 ( Table 2 , Figs 2c and 3a,c,e,g ). Indeed, the albedo change caused by simulated AF ( Table 3 , Supplementary Fig. 6b ) actually results in more warming (see text below for details) than if no climate engineering was implemented. SRM is the only method in our simulations that is potentially able to restore the temperature to a near pre-industrial value within the twenty first century ( Table 2 , Figs 2c and 3i ) and to prevent many warming-related Earth system changes from occurring ( Supplementary Figs 6i,j, 7i,j, 8j and 9e ). However, as already known from other studies employing different scenarios [28] , [29] , a persistent reduction of warming requires that SRM is applied continuously. Figure 3: Climate engineering method effects on temperature and carbon storage. The simulated year 2100 mean annual differences between the climate engineering runs and the control run (climate engineering run minus the control run) for surface air temperature ( a , c , e , g and i ) and terrestrial and oceanic carbon inventories ( b , d , f , h and j ). Note the difference in the surface air temperature scale for solar radiation management. Full size image Discontinuation of climate engineering If SRM is discontinued at any time then extremely rapid warming occurs (up to 0.36 °C y −1 ), along with an increased rate of atmospheric CO 2 accumulation ( Fig. 2b,d ; Supplementary Fig. 10 ). For temperature, this termination effect is well known and has been consistently reproduced in SRM studies [28] , [29] , [30] , [31] , [32] . However, there is much less certainty concerning the response of the carbon cycle to SRM discontinuation [30] . Here we show that there is a substantial termination effect on the carbon cycle since the reduction in atmospheric CO 2 , which for the simulated SRM deployment is even larger than that of the CDR methods ( Table 2 , Fig. 2a ), quickly reverses with atmospheric CO 2 levels reaching those of the control run within a few decades ( Fig. 2b ). For OU, rapid warming (up to 0.33 °C y −1 ) also occurs when it is discontinued, with surface air temperature ultimately becoming 0.24 °C higher, due to the method’s impacts on the planetary energy budget (see below and ref. 27 , than if the method had not been deployed at all. Atmospheric CO 2 concentrations also rise again with the discontinuation of OU until they are at essentially the same level as if no climate engineering had occurred. If the other methods are discontinued less dramatic changes occur. When OIF and OA are discontinued then the ocean stops taking up CO 2 at a higher rate ( Fig. 2b ; Supplementary Fig. 10 ). However, essentially all of the CO 2 that was taken up ( Fig. 3d,f ) remains in the ocean throughout the duration of the simulation and atmospheric CO 2 concentrations are 21 (OIF) and 48 (OA) p.p.m. lower in the year 2100 than if the methods had not been deployed at all. Because of this, surface air temperatures in the OIF and OA simulations always remain slightly lower, by 0.09 and 0.18 °C by the year 2100, respectively, than in the control run ( Fig. 2d ; Supplementary Fig. 10 ). For OIF, this result is consistent with an earlier study [26] . When AF is discontinued by stopping irrigation, the afforested desert regions eventually return to a desert state and the carbon that was stored in the plant biomass and soil ( Fig. 3b ) is slowly returned to the atmosphere through decay and respiration. As the vegetation related albedo change ends the surface air temperature drops from slight slightly higher (0.1 °C) to slightly lower (0.08 °C) than the control run ( Table 3 , Supplementary Fig. 6 ; see also text below), which is an effect that has been seen in other studies of deforestation [33] . The temperature becomes slightly lower than in the control run because atmospheric CO 2 is lower since not all of the stored carbon has returned to the atmosphere by the year 2100 and because during desertification the deserts expand (~1–3 model grid cells; not shown) beyond their former range (for example, the desert areas in the control simulation). Since more desert area increases the land surface albedo this contributes to the slight decrease in surface air temperature. The expansion of the deserts occurs because during simulated AF the vegetation in the grid cells next to the irrigated regions receive more water due to runoff and additional precipitation (see text below) and thus the vegetation changes from grass land (C3 and C4 types), as in the control simulation, to a shrub type. When simulated irrigation stops, the vegetation is unable to revert from a shrub type to grass types in our model world that has undergone climate change and instead becomes a desert. Similar shifts in vegetation have been observed in other simulations in response to perturbations [34] . Efficacy of the climate engineering methods Although most of the CDR methods ( Table 1 ) appear to gradually affect atmospheric CO 2 and the surface air temperature ( Fig. 2a,b ), their CDR efficacy is actually quite non-linear with time ( Fig. 4b–d ), and there is often a backflux of carbon from non-targeted areas as they adjust to the change in atmospheric CO 2 (for example, the ocean in the case of AF; backfluxes may also occur within the reservoirs). Indeed, even with SRM, whose purpose is to gradually reduce incoming solar radiation ( Fig. 4a ) to regulate the surface air temperature, the effectiveness-amplifying (in terms of surface air temperature reductions) CDR side effects (mainly on terrestrial productivity and soil respiration; see text below) are substantial ( Fig. 4b–d ; Supplementary Fig. 11 ). Some CDR methods like AF, OIF and OU are quite effective on short time scales (peak C removal occurs in the first 5 years), but less so on longer ones, a result that has been previously shown for OIF and OU [25] , [26] , [27] . In contrast, CDR for OA increases in effectiveness over time ( Fig. 4b–d ) because the ocean-buffering capacity [35] remains high, unlike in the other simulations, even as atmospheric CO 2 increases, thus allowing the ocean to take up more CO 2 . For SRM, CDR per change in insolation is highest during the first few years, then declines, and then gradually increases in intensity again ( Fig. 4b–d , Supplementary Fig. 11 ). The change in surface air temperature per change in insolation for SRM occurs mostly during the first decade of deployment ( Fig. 2c , Supplementary Fig. 11 ). These results highlight the non-linear relationship between changes in temperature and CO 2 , illustrated in Fig. 4d , that occur because of other, often method-specific, feedbacks involving, among others, the hydrological cycle, vegetation and ocean chemistry (see text below). 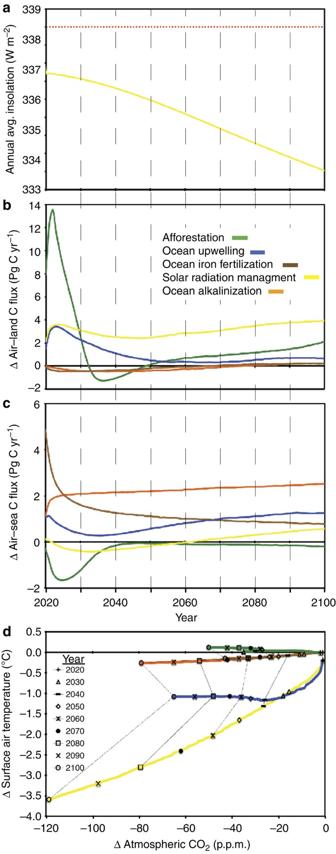Figure 4: Comparison of climate engineering method effectiveness. (a) Insolation at the top of the atmosphere for the SRM (yellow line) model run and all other simulations (dotted red line). The climate engineering model run differences (relative to the no climate engineering model run) in the annually averaged fluxes of carbon from the atmosphere to the (b) land and (c) ocean. Comparison (d) of surface air temperature versus atmospheric CO2differences (relative to the no climate engineering model run) for the climate engineering simulations. Figure 4: Comparison of climate engineering method effectiveness. ( a ) Insolation at the top of the atmosphere for the SRM (yellow line) model run and all other simulations (dotted red line). The climate engineering model run differences (relative to the no climate engineering model run) in the annually averaged fluxes of carbon from the atmosphere to the ( b ) land and ( c ) ocean. Comparison ( d ) of surface air temperature versus atmospheric CO 2 differences (relative to the no climate engineering model run) for the climate engineering simulations. Full size image Side effects of the climate engineering methods All of the methods have unintended side effects. Here we mainly focus on physical and biogeochemical side effects that can be diagnosed with the current model ( Tables 3 and 4 ), but we will also mention some other commonly discussed ones. When possible, we have tried to indicate whether a system or cycle will be perturbed by a side effect, but in most cases we are unable to make robust inferences on specific responses to a perturbation (for example, how species or small-scale regions may be affected). Table 4 Side effects of the climate engineering methods. Full size table The side effects of AF tend to be regional, with the large-scale regions defined here as N. Africa, Australia and the surrounding few hundred kilometres. However, although regional changes would certainly be expected, caution must be taken when interpreting the robustness of these results since the model has fixed atmospheric circulation patterns that essentially do not change (see methods) in response to AF. Regional precipitation and terrestrial productivity both increase ( Table 2 , Supplementary Figs 6a and 12a,c ), which could be beneficial for some species and, presumably, humans as long as the increase in precipitation does not cause severe storms or flooding. However, these changes would have a large and perturbing impact on local ecosystems and any societies that depend on them. Productivity increases because in addition to the direct effects of having more water from irrigation, which allows plants to grow in a former desert, there is the fertilizing effect of increasing CO 2 on growth [23] . Increasing CO 2 during the simulations has a further effect on vegetation and the hydrological cycle because vegetation water-use efficiency increases with increasing atmospheric CO 2 concentrations [22] , [23] , [36] . Although the increase in precipitation is regional it increases the total amount of global precipitation ( Fig. 2e ) because more water is added to the hydrological cycle. The higher soil moisture and precipitation, which also result in more terrestrial runoff into the ocean, thereby decrease coastal salinity ( Supplementary Fig. 7b ) and raise the global mean sea level by ~13 cm in the year 2100, unless the water used for irrigation is desalinated seawater. As a result of this change in salinity regional ocean circulation patterns ( Supplementary Fig. 8b ) and ecosystems would likely be affected as well. Increasing the amount of soil moisture also results in evaporative cooling ( Supplementary Fig. 8a ). However, this cooling is countered by a decrease in the regional surface albedo ( Supplementary Fig. 6b ) when the more reflective desert is replaced by darker vegetation. As a result the air temperature in the region increases ( Fig. 3a ) because of a sensible heat gain. Present-day AF simulations in boreal areas have produced similar albedo-related increases in temperature [37] . Another interesting, but not simulated, potential side effect of AF is that there would likely be less dust blown off of these desert regions if afforested (that is, both wind patterns and sources of dust may change). Since this dust contains iron and other nutrients that are known to fertilize the ocean [38] and distant forests such as the Amazon, it is possible that productivity in these regions could decrease [39] , [40] . Thus, an increase in productivity and carbon uptake in the afforested areas could result in a decrease in other areas, making this method potentially less effective as a carbon sink [40] . Both OU and OIF increase local marine productivity ( Table 3 , Supplementary Fig. 6e,g ), which may be beneficial for some species and fisheries [27] . However, the ecosystems of these fertilized regions (throughout the water column) would be disrupted by these changes [26] , [27] . Indeed, because of all the carbon that is locally sequestered and then respired during OIF, pCO 2 increases and the pH decreases more rapidly near Antarctica than in the control run ( Supplementary Fig. 13e,f ). Other OIF studies [26] have reported a similar result with regional declines in pH of up to 0.15 units (relative to a control run). A similar effect (pCO 2 increase, pH decrease) occurs during OU when sequestered carbon is upwelled, for example, in the tropical upwelling regions ( Supplementary Fig. 13g,h ). These methods also decrease productivity in some unfertilized regions because more nutrients are utilized before being transported out of the fertilized region [25] , [26] . Thus, non-local ecosystems and fisheries could also be affected. As has previously been shown for OIF [26] , it and OU increase ocean deoxygenation ( Fig. 2g ; Supplementary Fig. 9c,d ), due to the respiration (data not shown) of fertilization-induced organic matter in deeper waters. As a result the size of suboxic (O 2 <10 μM) regions changes ( Supplementary Fig. 4 ), impacting marine ecosystems and biogeochemical cycles [26] , [27] . The simulated 265% increase in the size of the suboxic zones caused by OU may be particularly important because it could have climatic feedbacks due to the production of methane and N 2 O, which are potent greenhouse gases, in low-oxygen waters [27] , [41] . Although the overall percent fraction that is suboxic with OIF decreases by 43% because of less productivity, export and respiration outside of the fertilized area [26] , oxygen declines in the Southern Ocean in our model ( Supplementary Fig. 9c ), with some regions becoming suboxic by the year 2125. This OIF-induced oxygen decline is much stronger than in an earlier OIF modelling study [26] that found only minor decreases in oxygen (60 mmol m −3 ) in the Southern Ocean by the year 2110. Since most of the oxygen is consumed in deeper waters that will not be at the surface, where air–sea gas exchange can occur, for tens to hundreds or thousands of years, discontinuing OIF and OU does not restore oxygen to the state that it is in the control simulation ( Fig. 2h ). For OU there are also a number of simulated side effects related to the cooling of the Earth’s surface. Terrestrial productivity is perturbed and in most places there is less soil respiration ( Table 3 , Supplementary Figs 6g and 9h ), which together results in more terrestrial C storage ( Fig. 3h , Table 2 ). However, unlike in an earlier OU study [27] where 80% of sequestered C was stored in the terrestrial system by the year 2100, only 54% was in our study, which can be explained by the consideration of iron limitation and iron upwelling in our study (see Methods). Precipitation patterns are also altered ( Supplementary Fig. 12g,h ), with a decrease in total precipitation ( Fig. 3e , Table 3 ) because of decreases in evaporation and evapotranspiration [28] . In addition, as in an earlier study [27] , OU decreases sea-ice loss and perturbs ocean temperature, salinity, stratification and circulation ( Supplementary Figs 7g,h, 8g,h and 14b ). Together, these side effects alter the planet’s heat-budget and cause the Earth to take up additional heat and store it in the ocean’s low-latitude subsurface waters ( Supplementary Fig. 14b ; see ref. 27 for further details). As a result this method cannot be stopped without causing rapid warming that ultimately exceeds that of the control run [27] ( Fig. 2d ). OA has few side effects that can be diagnosed with our model. The ones that we can diagnose reduce the rate of ocean acidification ( Supplementary Fig. 13d ) and keep the saturation states of aragonite and calcite higher than with most other methods ( Table 3 ), despite higher oceanic carbon uptake ( Fig. 3d , Table 2 ). However, other studies have noted that there are likely to be other side effects that impact marine ecosystems [24] , [42] and shown that certain species physiology would be altered by OA [43] . Furthermore, this method is also likely to have a substantial impact on terrestrial systems due to the mining and production process associated with the alkalizing agent [24] , [42] . For SRM there are a number of side effects related to the cooling of the Earth’s surface. Terrestrial and marine productivity are perturbed and there is less soil respiration ( Table 3 , Supplementary Figs 6i and 9j ), which ultimately results in more terrestrial C storage ( Table 2 ). For global terrestrial NPP, which is 1.7 Pg C y −1 higher in the year 2100 than in the control run, this increase is consistent with other SRM studies (for example, in the GeoMIP G1 experiments the model’s mean change in NPP between the SRM runs and the quadrupled CO 2 control runs was 1.8 Pg C y −1 ) [44] , [45] . Interestingly, this accumulation of C on land decreases surface-ocean pCO 2 and reduces the rate of ocean acidification ( Table 3 , Supplementary Fig. 13i,j ). Precipitation patterns are also altered, with a decrease in total precipitation ( Fig. 3e ; Table 3 , Supplementary Fig. 12i,j ), because of less evapotranspiration [28] and evaporation [22] , [46] . Other studies [22] , [28] , [44] , [47] have found a similar decrease in precipitation when SRM is implemented. However, since evapotranspiration in our model is more sensitive to CO 2 increases than in other models and precipitation is simulated with a simple energy–moisture balance model, we performed the GeoMIP G1 experiment [48] to gain a better understanding of how this particular result compares with other SRM experiments. This experiment (G1) involves instantaneously quadrupling the CO 2 concentration (from pre-industrial levels) while simultaneously reducing the solar constant to counteract this forcing (50-year simulation). In this experiment we found that global precipitation decreased by 0.26 mm d −1 (a 9% reduction), which is more than the mean 0.1 (range: 0.1–0.2) mm d −1 decrease (a mean reduction of 4.5%) found with the GeoMIP models [44] . While this appears to be a substantial difference, when we spatially compare the results of last 10 years of our G1 simulation with the results from one of the GeoMIP models (MPI-ESM-LR), which has itself been comparatively assessed [44] , we are able to discern that the regional changes are higher in the MPI-ESM-LR even though the global mean effect is smaller ( Supplementary Fig. 15 ). Thus, these GeoMIP model results actually indicate that larger, more extreme SRM-induced changes in regional tropical precipitation are possible, even if the global mean change is less than in our simulations. These differences likely reflect the differences in the atmospheric model components (for example, UVic’s simple atmosphere versus the more complex, higher resolution one in the MPI-ESM-LR). Another important side effect is that CO 2 continues to accumulate and therefore SRM cannot be discontinued without causing rapid global change [28] , [29] , [30] ( Fig. 2 , right panels). The C stored mostly in the soils during the deployment of SRM is released rapidly once temperatures increase. Finally, there are also likely to be other side effects beyond what we can diagnose, as other studies have indicated that if SRM is aerosol-based it will potentially affect atmospheric chemistry by depleting the ozone layer [49] and altering the optical properties of the sky (that is, colour, whiteness) [2] . Furthermore, chemical-aerosol altering interactions may occur and reduce the method’s effectiveness [49] . As discussed in other studies [3] , [5] , [28] , [46] , [49] , these side effects, especially in the case that SRM is discontinued, could severely disrupt ecosystems and human societies. While the effectiveness and the consequences of discontinuing the methods have, for some methods, been studied before [3] , [30] and evaluated and ranked in comparative frameworks [3] , [4] , [5] , this study for the first time uses an Earth system model for a comparative evaluation of the effectiveness of the different schemes. Unlike in previous studies, we thereby have been able to compare many of the side effects associated with the methods ( Table 4 ) in a quantitative manner ( Table 3 ). However, our study does have its limits. Foremost, our experiments were conducted with a single model for a limited number of idealized methods. Since every model has its own particular deficiencies and is only as good as its assumptions, further research with other models and scenarios is required. Model intercomparison projects such as GeoMIP [48] and model uncertainty analyses, both individual and multi-model, will also be necessary to achieve a high level of confidence in the results. More methods may also need to be included in these evaluations, along with possible combinations of methods (for example, SRM and OA) and mitigation efforts (for example, SRM and carbon capture and storage). Another aspect that needs to be considered is that while we do discuss large-scale regional effects, these results are likely to be less robust than the global-scale ones due to the coarse resolution of our model. Therefore, future climate engineering studies should also be conducted with less heavily parameterized, higher resolution models to investigate regional effects. Furthermore, since these experiments were designed to evaluate what we deemed near-maximum effects, they did not consider any practical realities of deployment, which would have to be taken into account as the research becomes more focused. Whether or not the magnitude (effectiveness) of the methods can be more than what we decided was optimistically feasible must be considered in future research. To further increase AF efficacy the forests could be better managed (that is, the careful husbandry of selected optimal species or even of genetically engineered species with the vegetation periodically harvested and the C biomass permanently removed from the active C cycle). More large-scale forests could also be planted, although this would likely bring AF into competition with existing areas of food production. For OIF, there is likely little that can be done to increase efficacy as a previous study [25] found that fertilizing the areas outside of the Southern Ocean results in a negligible amount of carbon sequestration. For OU, the pipe location selection criteria (see ref. 27 ) could be modified to include iron and nitrate limitation or non-Redfield nutrient uptake. This would mostly result in the placement of pipes in the Southern Ocean, which is the major area where pipes currently aren’t placed. Since nutrients are already plentiful here the increase in efficacy would be similar to that of OIF, but with the additional side effects of OU. For OA, the CDR efficacy could theoretically be increased if production and transport logistics, which we used to constrain this method, allow more of the alkalizing agent to be added to the ocean [50] . However, any increase would take time since shipping and production capacity would need to be built up. Given the limited effectiveness of the CDR methods in our study, even with our optimistically large deployments, a very substantial increase in the magnitude (efficacy) mentioned above would be needed to make much of a difference. However, for SRM, insolation could have been reduced more rapidly with our idealized methodology than in Fig. 4a (that is, as in other SRM experiments when it is deployed later in the twenty first century to counter higher temperatures [28] , [51] ), although there would be no reason to do so unless temperatures below pre-industrial levels were desired. Moreover, from a practical standpoint there are some legitimate concerns that have been discussed in other studies [3] , [49] about the practical logistics of aerosol deployment or other SRM methods. In summary, our study suggests that even if continuously deployed on a massive scale, the evaluated CDR-based methods are able to only sequester an amount of atmospheric CO 2 that is small compared with cumulative anthropogenic emissions in the RCP 8.5 scenario and are thus unable to prevent the mean surface temperature from increasing to well above 2 °C by the year 2100 ( Figs 2a,c and 3 ; Table 2 ). This is a result that holds true even if the methods that can be safely stopped (AF, OIF and OA) are combined ( Table 2 ; Supplementary Fig. 16 ). SRM is the method that has the largest potential for preventing warming and even for sequestering carbon, which is an effectiveness-amplifying side effect. However, SRM also has some of the largest side effects and cannot be discontinued without causing rapid climate change ( Fig. 2 ; Supplementary Figs 6i, 10 and 12 ). Together, these results suggest that if CO 2 emissions remain high, the climate engineering methods discussed here should not be solely counted on to prevent warming or large-scale changes to the Earth system. Indeed, given the limited effectiveness of most of the evaluated methods, our results suggest, in agreement with other studies [3] , that CO 2 emission mitigation seems the most effective way to prevent climate change. Climate engineering does not appear to be an alternative option, although it could possibly be used to compliment mitigation [3] . However, if climate engineering is seriously considered as one of the means of preventing climate change, care must be taken when evaluating whether the potential reductions in atmospheric carbon and temperature of a particular method are worth the risks and costs of its side effects. Model description The model (UVic version 2.9) consists of three dynamically coupled components: a three-dimensional (3D) general circulation model of the ocean that includes a dynamic–thermodynamic sea-ice model, a terrestrial model and a simple one-layer atmospheric energy–moisture balance model. All components have a common horizontal resolution of 3.6° longitude × 1.8° latitude. The oceanic component, which is in the configuration described in ref. 8 , has 19 levels in the vertical with thicknesses ranging from 50 m near the surface to 500 m in the deep ocean. The terrestrial model of vegetation and carbon cycles [52] is based on the Hadley Center model TRIFFID. The atmospheric energy–moisture balance model interactively calculates heat and water fluxes to the ocean, land and sea ice. Wind velocities, which are used to calculate the momentum transfer to the ocean and sea-ice model, surface heat and water fluxes, and the advection of water vapour in the atmosphere, are determined by adding wind and wind stress anomalies (as determined from surface pressure anomalies that are calculated from deviations in pre-industrial surface air temperature) to prescribed NCAR/NCEP monthly climatological wind data [53] . The model has been extensively used in climate change studies and is also well validated under pre-industrial to present-day conditions [7] , [8] , [9] , [10] , [54] . Experimental design The model was spun up for 10,000 years under pre-industrial atmospheric and astronomical boundary conditions and then run from 1765 to 2000 using historical fossil fuel and land-use carbon emissions. From the year 2000 to 2100 the model was forced with CO 2 emissions following the Representative Concentration Pathway (RCP) 8.5 scenario, which is a ‘business-as-usual’ high CO 2 emission scenario [6] . Continental ice sheets, volcanic forcing and astronomical boundary conditions were held constant to facilitate the experimental set-up and analyses (that is, prevent confounding feedback effects). Supplementary Figs 1–3 show the ‘control’ run results. Simulated climate engineering ( Table 1 ) starts in year 2020 and is either applied continuously until the year 2100 or stopped after 1, 10 and 50 years, with the runs continuing thereafter until year 2100 ( Fig. 1 ). All methods, except for SRM and OU, are instantaneously deployed and stopped at full scale. Simulated AF The simulated AF of North Africa (the Sahara desert) and the Australian Outback is based on a previous study [39] , which we have chosen to replicate because this avoids conflicts with current food production, even though it requires expensive large-scale irrigation measures. Irrigation is simulated by forcing the soil moisture to have a constant value of 360 kg m −2 ( Supplementary Fig. 17 ), which then allows vegetation to grow and remove CO 2 from the atmosphere. The irrigated regions were chosen to replicate the previous experiment [39] and we refer readers to this article for justification of the chosen locations. In our simulations only the direct effects of AF on carbon uptake, surface albedo and the energy–moisture balance are considered. The frictional effect on winds is not investigated, nor is the potential limitation of vegetative growth by nutrients other than carbon. The possible reduction of desert dust transport and deposition are not considered here either and will be further investigated elsewhere. Simulated OU Simulated OU was based on a previous study with the UVic model [27] . This method places ‘pipes’ that pump water from the specified lower end of the pipe (up to 1,000 m deep) to the ocean surface, in areas where upwelling has been calculated to reduce surface-ocean pCO 2 ( Supplementary Fig. 14a ). The simulated upwelling works by transferring water adiabatically from the grid box at the lower end of the pipe to the surface grid box at a rate of 1 cm d −1 . A compensating downwelling velocity at all intermediate levels insures volume conservation. The modelled pipes operate at any water column at any time for which a pipe-induced local reduction in surface pCO 2 can be expected (included in this calculation is the assumption that surface phosphate concentrations are <0.4 mmol m −3 so that a fertilization effect occurs). In contrast to the previous study [27] , the ecosystem model now includes phytoplankton iron limitation [8] and the method was modified so that iron is not limiting in the grid cells where the pipes are located. This implementation relies on the assumption that either there is bioavailable iron at the depths from which the pipes draw water or that particle-bound iron is desorbed and becomes bioavailable when it is pumped to the surface. Observations [55] indicate that in ocean regions where dust deposition is low, dissolved iron concentrations are higher at depth than at the surface, suggesting that artificially upwelling these waters will increase surface iron concentrations. Since bioavailable iron is quickly utilized or abiotically scavenged [38] , [55] it was also assumed that upwelled dissolved iron is removed before it can be exported to adjacent grid cells. Simulated OA OA by Ca(OH) 2 addition was simulated by evenly increasing the total alkalinity of surface waters between 70° N and 60° S (that is, in ice-free waters accessible throughout the year) ( Supplementary Fig. 18 ). The premise behind this method is that the addition and dissolution of Ca(OH) 2 in seawater increases the total alkalinity and thereby removes CO 2 from seawater in the following reaction: As a result of (1) the ocean takes up more CO 2 due to the conversion of CO 2 to HCO 3 − at a molar ratio of 2 moles per added mole of Ca(OH) 2 . Equation (1) also implies that for every mole of Ca(OH) 2 added total alkalinity increases by 2 moles. Since limestone, from which Ca(OH) 2 is derived, is readily abundant the major limits are either those of production or the capacity to deliver it. The amount we added, 10 Pg y −1 , is based on another study [24] , which estimated that the total transport capacity of all large cargo ships and tankers is ~10 Pg y −1 . Our simulation of OA may thus be viewed as of maximum intensity based on current transport capacity. Simulated OIF To simulate the maximum potential of OIF we followed previous studies [26] , [56] and focused on the Southern Ocean as the region with the largest carbon sequestration potential by OIF because it has the largest inventory of unused surface macronutrients, has been identified as being iron limited [57] , [58] and is a site of large water-mass transformations [59] , [60] , which help to keep regionally exported carbon in the ocean’s interior. Furthermore, Southern Ocean surface pCO 2 drawdown and deep carbon export has been observed during iron fertilization experiments [61] , [62] and simulated by modelling studies [25] , [26] . Our simulated Southern OIF works in an idealized manner by simply releasing phytoplankton from iron limitation everywhere south of 40°. Simulated SRM There is, so far, little information about the maximum possible intensity of SRM. In this study we set the intensity of SRM such that SRM restores and maintains near pre-industrial atmospheric temperatures. The methodology is based on previous SRM simulations with the UVic model [28] and works by reducing the radiative forcing in the model ( Fig. 4a ) to mimic what would happen if hypothetical SRM techniques, such as the stratospheric injection of reflective aerosols or space-based sunshades [3] , were successfully deployed. As in a previous study [28] SRM is represented by applying a factor, K g , during each time step to incoming solar radiation (the solar constant), , before the incoming shortwave radiation at the top of the atmosphere; S C , is calculated for each grid cell so that and In (3) F is the atmospheric CO 2 radiative forcing term [53] and has a constant value of 5.35 W m −2 , CO 2 is the simulated atmospheric CO 2 concentration, and χ CO 2 , which equals 280 p.p.m., is the atmospheric CO 2 concentration that corresponds to the target radiative forcing, and α P equals 0.7, which is approximately one minus the globally averaged planetary albedo. How to cite this article: Keller, D. P. et al . Potential climate engineering effectiveness and side effects during a high CO 2 -emission scenario. Nat. Commun. 5:3304 doi: 10.1038/ncomms4304 (2014).